Discovery of X-ray pulsations from a massive star X-ray emission from stars much more massive than the Sun was discovered only 35 years ago. Such stars drive fast stellar winds where shocks can develop, and it is commonly assumed that the X-rays emerge from the shock-heated plasma. Many massive stars additionally pulsate. However, hitherto it was neither theoretically predicted nor observed that these pulsations would affect their X-ray emission. All X-ray pulsars known so far are associated with degenerate objects, either neutron stars or white dwarfs. Here we report the discovery of pulsating X-rays from a non-degenerate object, the massive B-type star ξ 1 CMa. This star is a variable of β Cep-type and has a strong magnetic field. Our observations with the X-ray Multi-Mirror (XMM-Newton) telescope reveal X-ray pulsations with the same period as the fundamental stellar oscillations. This discovery challenges our understanding of stellar winds from massive stars, their X-ray emission and their magnetism. Massive stars ( M initial ≳ 8 M ⊙ ) are among the key factors in the cosmic evolution. These stars generate most of the ultraviolet radiation of galaxies and power their infrared luminosities. Massive stars and their final explosion as supernovae provide significant input of radiative and mechanical energy into the interstellar medium, inject nuclear processed material and largely drive the evolution of star clusters and galaxies. All hot massive stars drive stellar winds by their intense radiation [1] . Photons that are scattered or absorbed in spectral lines transfer their momentum and thus accelerate the matter to highly supersonic velocities, typically of the order of 1,000 km s −1 . This driving mechanism is unstable [2] . It is generally believed that the wind instability may result in shocks where part of the wind material is heated to X-ray-emitting temperatures. These wind shocks are often invoked to explain the thermal X-ray emission, which is ubiquitously observed from massive stars [3] . A small fraction of massive stars, including some B-type stars, possess strong, large-scale magnetic fields [4] . According to one hypothesis, such stars may have undergone a recent merger process, which powered a dynamo mechanism [5] . Strong magnetic fields can significantly influence the dynamics of stellar winds [6] . If the magnetic field has a dipole configuration, the strong field can in effect channel the wind towards the magnetic equator, where the wind streams from the opposite hemispheres collide. The formation of a strong stationary shock is predicted, and it is expected that the X-ray properties of stars with strong magnetic fields will be different from those of non-magnetic stars, for example, the X-ray temperatures for magnetically confined winds should be higher [7] . The two models briefly outlined above (embedded wind shocks for non-magnetic objects and magnetically confined winds) are widely adopted to interpret the X-ray emission from single hot massive stars. However, neither of these models accounts for the effects of stellar oscillations. The majority of all massive stars are of spectral types B0–B2 with effective temperatures T eff >15,000 K. These stars were born with masses between 8 and 18 M ⊙ . While still young and burning hydrogen in their cores, B0–B2 type stars oscillate with periods of a few hours. The physical mechanism that drives these oscillations is well understood and is attributed to changes in the opacity within the star during the pulsation cycle ( κ -mechanism) [16] . A whole class of such variables is termed after its prototype β Cephei. The object of our study, ξ 1 CMa (alias HD 46328, HR 2387 and HIP 31125), belongs to this class. 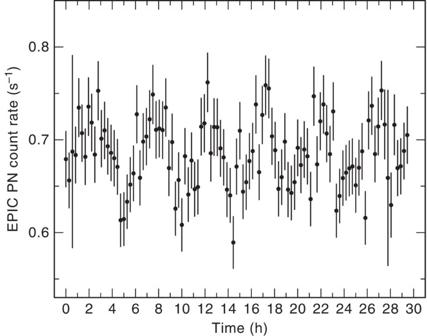Figure 1:X-ray light curve of ξ1CMa. Data are for the 0.2–10.0 keV (1.24–62 Å) energy band, where the background was subtracted. The horizontal axis denotes the time after the beginning of the observation in hours. The data were binned to 1,000 s. The vertical axis shows the count rate as measured by the EPIC PN camera. The error bars (1σ) correspond to the combination of the error in the source counts and the background counts. A summary of its stellar parameters is provided in Table 1 . The variability of ξ 1 CMa has been known for more than 100 years [17] . Its photosphere oscillates radially with a velocity amplitude Δ υ rad =34.2±0.7 km s −1 that exceeds the local speed of sound [18] , [19] , which is rare among β Cep variables. Together with the radial-velocity variations, the star shows periodic photometric variability in visual light. Maximum light occurs about 25 min after minimum radius [18] . The amplitude of photometric variability increases strongly with decreasing wavelength; in the ultraviolet near λ= 1,550 Å it amounts to 0.161 mag [20] . Table 1 Parameters of ξ 1 CMa. Full size table ξ 1 CMa shows remarkable stability of its pulsational behaviour: its period is constant to about 1 s per century [18] . The pulsations are nonlinear and monoperiodic, with only one frequency and its first harmonic being significant [21] , [19] . The fundamental stellar parameters of ξ 1 CMa are typical for its spectral type. The effective temperature changes by Δ T eff =1,000 K over the pulsation cycle, while log g changes between 3.7 at maximum and 3.8 at minimum [9] . Similar to some other magnetic early B-type stars, nitrogen is overabundant by a factor of 3-4 in ξ 1 CMa as compared with the solar value [9] . The advent of ultraviolet spectroscopy provided evidence for a stellar wind from ξ 1 CMa [22] , [23] . The stellar wind parameters of ξ 1 CMa were constrained from the analysis of ultraviolet spectral lines by means of non-local thermodynamic equilibrium iron-blanketed model atmospheres calculated with the Potsdam Wolf-Rayet (PoWR) code [24] . X-rays have a strong effect on the ionization structure of the cool wind component [11] . Despite earlier attempts [25] , the first firm detection of a magnetic field on ξ 1 CMa was achieved only recently [13] . Among pulsating B-type stars with known magnetic fields, ξ 1 CMa has by far the strongest field with a polar strength of ∼ 5 kG. The longitudinal magnetic field shows periodic modulations with a period of ≈2.2 days. This period is identified with the stellar rotation. The rotational velocity of ξ 1 CMa is established as υ sin i =9±2 km s −1 from fitting its high-resolution optical spectrum [10] . From this value of υ sin i and the rotation period it follows that the inclination is very small ( i ≈3°), that is, we look almost exactly at the star’s rotational pole. The spectropolarimetric observations are best explained by assuming that the axis of the magnetic field is inclined by about 79° to the rotation axis; consequently, we have a nearly constant edge-on view of the system’s magnetic equator. The field has a dipole geometry, albeit additional magnetic structures on smaller spatial scales cannot be excluded [12] . The first X-ray survey of β Cep-type stars was performed by the Einstein observatory [26] . ξ 1 CMa was detected as the most X-ray luminous star in this survey [26] , [27] . First X-ray spectra were obtained with the Rosat observatory. It was found that the X-ray spectrum of ξ 1 CMa is somewhat harder than of other B-type stars [28] . In this work we report sensitive X-ray observations of ξ 1 CMa with the XMM-Newton observatory. Their analysis reveals X-ray pulsations that are in phase with the optical light curve. The high-resolution spectra show phase-dependent variability. The phase-resolved spectra provide indications of higher X-ray temperatures in the minimum than in the maximum. Current models of stellar winds and magnetic massive stars do not provide explanations to the observed X-ray pulsations. Observations with the X-ray multi-mirror satellite The X-ray data for ξ 1 CMa discussed in this paper were taken with the X-Ray Multi-Mirror Mission XMM-Newton of the European Space Agency ESA. Its three telescopes illuminate five different instruments, which always operate simultaneously and independently: RGS1 and RGS2 are reflection grating spectrometers [29] , achieving a spectral resolution of ∼ 0.07 Å in the wavelength range 5–38 Å. The other three focal instruments, forming together the EPIC camera, are called MOS1 and MOS2 (metal-oxide semiconductor) and PN (pn-CCDs). Compared with the RGSs, the EPIC instruments have a broader wavelength coverage of 1.2–60 Å, but their spectral resolution is much lower ( E /Δ E ≈20–50) [30] , [31] . In addition to X-ray telescopes, XMM-Newton has also an optical monitor. However our target is too bright in visual light to be observed with the optical monitor. The first dedicated XMM-Newton observation of ξ 1 CMa started on 3 September 2009 with an exposure time of 2 h, which was far too short to reveal the periodic variability [11] . In October 2012, XMM-Newton continuously observed ξ 1 CMa during nearly 29 h (Unique Observation Identifier 0600530101). The light curves and spectra were recorded by all X-ray instruments. The sensitivity of the PN camera is superior, and therefore its data are best suited for time-variability studies. The data reduction involved standard procedures of the XMM-Newton Science Analysis System (SAS) v.13.0.1. The event lists have been filtered, and time intervals affected by high background were excluded. The object of our study is sufficiently isolated, with no nearby bright optical or X-ray sources. Because of the brightness of the target in the visual, the optical light-blocking filter of XMM-Newton was used in its thick mode for our observations. We carefully investigated the potential contamination of the signal by optical/ultraviolet light. For the XMM-Newton detectors operating in full-frame mode and with the thick filter, no optical loading is expected for stars with m V >−1 to 2 mag (for the PN camera) and m V >1 to 4 mag (for the MOS cameras) (XMM-Newton User Handbook). Moreover, the optical loading would affect the softest part of the X-ray spectrum only, but we do not see different pulsational behaviour between softer and harder parts. Also, the amplitude of the pulsations is higher in the X-ray band than in the optical. From these considerations, a contamination of the signal by optical/ultraviolet light is ruled out. X-ray light curve and comparison with optical light curve Already visual inspection of the X-ray light curve reveals the periodic variability. Figure 1 shows the light curve of ξ 1 CMa in the energy band 0.2–10.0 keV (1.24–62 Å) where the background was subtracted. To quantify this variability, a statistical analysis is performed. To obtain a characterization of the variability, the light curves in three energy bands (total: 0.2–10.0 keV (1.24–62 Å); soft: 0.2–1.0 keV (12.4–62 Å); and hard: 1.0–10.0 keV (1.24–12.4 Å)) are extracted from the event lists of all three EPIC instruments separately. This is done using the SAS’s task EPICLCCORR, which provides equivalent on-axis, full-point spread function count rates with background correction. The data are binned in temporal bins of different duration (100, 500, 1,000, 3,600 s, see Figs 1 , 2 , 3 ). Figure 1: X-ray light curve of ξ 1 CMa. Data are for the 0.2–10.0 keV (1.24–62 Å) energy band, where the background was subtracted. The horizontal axis denotes the time after the beginning of the observation in hours. The data were binned to 1,000 s. The vertical axis shows the count rate as measured by the EPIC PN camera. The error bars (1 σ ) correspond to the combination of the error in the source counts and the background counts. 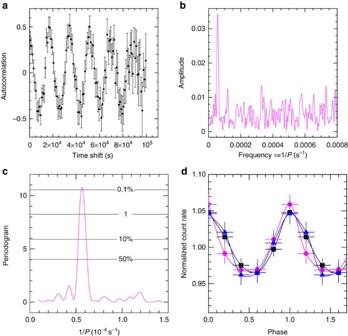Figure 2: Various statistical tests. (a) Result from an autocorrelation test for the PN light curve (with 1,000 s binning) in total band. Note that the point with zero shift is not shown. Error bars denote 1σdispersions of autocorrelation function estimates in individual time bins. (b) Fourier periodogram32,33for PN light curve (with 100 s binning). The associated spectral window is clean, the signal is therefore not spurious. (c) Power-density spectrum based on the Fourier transform34,35of the PN data. The periodogram was calculated fromν=1/Ptoν=N0/Pwith a spacingP−1, whereN0is the number of data points. Various false-alarm probability levels are marked; (d) EPIC PN light curves in full (black squares), in the soft (magenta dots) and in the hard (blue triangles) band folded with the Hipparcos ephemeris. The solid lines show a cubic spline interpolation. Horizontal bars show the bin size of Δφ=0.1. Vertical bars show 1σerrors. Full size image Figure 2: Various statistical tests. ( a ) Result from an autocorrelation test for the PN light curve (with 1,000 s binning) in total band. Note that the point with zero shift is not shown. Error bars denote 1 σ dispersions of autocorrelation function estimates in individual time bins. ( b ) Fourier periodogram [32] , [33] for PN light curve (with 100 s binning). The associated spectral window is clean, the signal is therefore not spurious. ( c ) Power-density spectrum based on the Fourier transform [34] , [35] of the PN data. The periodogram was calculated from ν =1/ P to ν = N 0 / P with a spacing P −1 , where N 0 is the number of data points. Various false-alarm probability levels are marked; ( d ) EPIC PN light curves in full (black squares), in the soft (magenta dots) and in the hard (blue triangles) band folded with the Hipparcos ephemeris. The solid lines show a cubic spline interpolation. Horizontal bars show the bin size of Δ φ =0.1. Vertical bars show 1 σ errors. 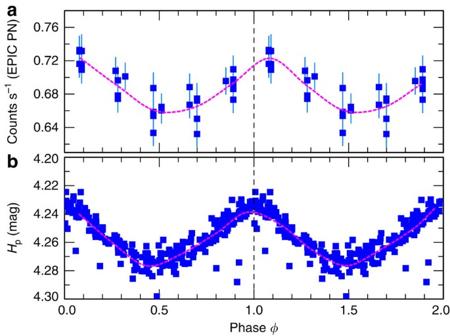Figure 3:Light curves of ξ1CMa phased with the Hipparcos ephemeris. (a) The X-ray light curve in the 1.2–62 Å band produced from the data obtained with the XMM-Newton EPIC PN camera, using 1 h binning. The X-ray data are background subtracted, and the error bars (1σ) reflect the combination of the statistical errors in the source counts and the background. The dashed magenta line interpolates the averages in phase bins of Δφ=0.1. (b) The Hipparcos Catalogue Epoch Photometry data. The abscissa is the magnitudeHpin the Hipparcos photometric system (330–900 nm with maximum at ≈420 nm). The dashed magenta line interpolates the averages. Full size image Figure 3: Light curves of ξ 1 CMa phased with the Hipparcos ephemeris. ( a ) The X-ray light curve in the 1.2–62 Å band produced from the data obtained with the XMM-Newton EPIC PN camera, using 1 h binning. The X-ray data are background subtracted, and the error bars (1 σ ) reflect the combination of the statistical errors in the source counts and the background. The dashed magenta line interpolates the averages in phase bins of Δ φ =0.1. ( b ) The Hipparcos Catalogue Epoch Photometry data. The abscissa is the magnitude H p in the Hipparcos photometric system (330–900 nm with maximum at ≈420 nm). The dashed magenta line interpolates the averages. Full size image We employ a χ 2 -test for several hypotheses such as constancy, linear variation and quadratic variation [36] . The PN and MOS1 data in soft and total bands display significant variations for all time binnings—the probability that the observed curve occurs by chance is <0.01. The autocorrelation test reveals periodic variability with a period of about 4.8 h (see Fig. 2a ). A Fourier algorithm [32] , [33] yields the period P =4.90±0.09 h with significance P <2 × 10 −8 (see Fig. 2b ). The power-density spectrum calculated with an alternative Fourier algorithm [34] , [35] gives a period of P =4.91±0.05 h with a false-alarm probability of F = 6.7 × 10 −4 (see Fig. 2c ). Hence, all these different methods provide consistent values for the X-ray pulsation period. To quantify the amplitude of the X-ray pulsations, we fit the X-ray light curve with a sinusoidal function and estimated the errors. In the full X-ray band, the peak-to-peak relative amplitude is 9.1±1.2%. Simultaneous optical and X-ray observations of ξ 1 CMa are not available. In order to investigate the phase correlation between X-ray and optical pulsations, we searched for optical photometric data in the archives. The best and most recent photometry of ξ 1 CMa was obtained by the space telescope Hipparcos during the years 1990–1993. The Hipparcos photometry was carried out in a wide pass-band, referred to as H p (ref. 15 ). All H p photometric data were analysed in a uniform and self-consistent manner and yielded the parameters of variability, which are compiled in the ‘Hipparcos Catalogue Epoch Photometry Data’ [14] . On the basis of the 5,482 observed cycles, the derived period is P =0.209577±0.000001 days and the epoch of zero phase is JD(TT) 2448500.0280. We retrieved the Hipparcos photometric data for ξ 1 CMa and folded them according to the Hipparcos ephemeris. The result is shown in Fig. 3b . Comparing this ephemeris to older measurements from 1954 (ref. 37 ), the light curve is found to be still in phase, that is, the period derived from Hipparcos photometry is precise and the pulsations have been stable over 40 years. The peak-to-peak variability in the optical light is only 3% relative to the median amplitude, that is, lower than in the X-ray light. The optical and X-ray period agree within 3 σ of the X-ray period. Our XMM-Newton data were obtained about 34,000 pulsation cycles after the Hipparcos measurements. However, given the stability of the ξ 1 CMa light curve [18] , the Hipparcos ephemeris can be meaningfully applied for the epoch of our X-ray observations. The X-ray light curves were phased with the Hipparcos ephemeris and compared with the optical ones as illustrated in Fig. 3a,b . The X-ray light curves turned out to be in phase with the optical within the precision of the measurement and the formal error margin of the ephemeris. Figure 2d shows the X-ray light-curves in the full, hard, and soft band, folded with the Hipparcos ephemeris. Typically, the optical light curve of β Cep-type variables is similar in shape to the radial-velocity curve but lags in phase. The maximum brightness occurs shortly after the stellar radius goes through its minimum. The results of our analysis show that the same is true for the X-ray light—the maximum X-ray brightness is observed close to the phase when the stellar radius is at its minimum. Analysis of the low-resolution X-ray spectra To define the physical properties of the X-ray-emitting plasma in ξ 1 CMa, we analyse its X-ray spectra. As a first step, the low-resolution data recorded by the EPIC cameras [30] , [31] are considered. While individual lines, in general, cannot be resolved with the EPIC, the low-resolution spectra cover a broad energy band and allow to constrain the temperature and the emission measure of the hot plasma. For a phase-resolved analysis, the spectra are extracted for time intervals close to the pulsation maximum and the pulsation minimum, respectively. The spectra are analysed with the standard spectral fitting software XSPEC [38] . The spectra were investigated for the presence of an emission component described by a power law. No convincing evidence for non-thermal radiation was found. Therefore, we adopted a model of optically thin thermal plasma in collisional ionization equilibrium as implemented in the apec code [39] . The most important parameters of this model are the electron temperature and the volume emission measure of the plasma. We follow here the definition of volume emission measure as used in the apec code, namely as the volume integral EM =∫ V N e N H d V , where N e and N H are the electron and hydrogen number densities, respectively. To restrict the number of free parameters, we use only three temperature components. Albeit such a model provides only a simplified description of the plasma, it can give insight in the characteristic temperatures and emission measures. Considering first the X-ray spectra obtained over the full exposure time, we fit the MOS and PN spectra simultaneously (see Fig. 4 ). The best fit resulted in a nitrogen overabundance by a factor of 4.3±0.8 relative to solar [40] , and an oxygen overabundance by a factor of 1.6±0.3. These abundances are in agreement with those found from the analysis of optical spectra of ξ 1 CMa [41] . 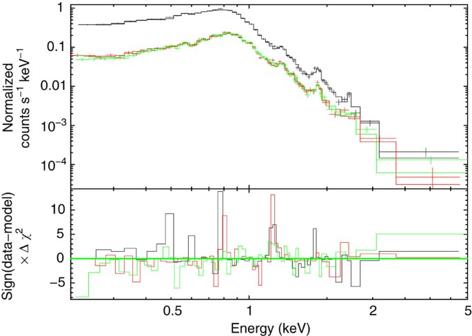Figure 4:Low-resolution X-ray spectra of ξ1CMa. The EPIC PN (black data points), MOS1 (red data points) and MOS2 (green data points) spectra integrated over the full exposure time are displayed. The black, red and green histograms show the best fit model of a three-temperature plasma and the residuals as signed contributions toχ2. Figure 4: Low-resolution X-ray spectra of ξ 1 CMa. The EPIC PN (black data points), MOS1 (red data points) and MOS2 (green data points) spectra integrated over the full exposure time are displayed. The black, red and green histograms show the best fit model of a three-temperature plasma and the residuals as signed contributions to χ 2 . Full size image The best spectral fit is obtained with N H =1.3 × 10 20 cm −2 with a 3 σ interval from 1 × 10 19 to 3 × 10 20 cm −2 . This can be compared with the interstellar reddening E B−V =0.04 mag that was estimated from fitting the observed spectral energy distribution of ξ 1 CMa from the ultraviolet to the optical [11] . Given the range of conversion factors from reddening to neutral hydrogen column density as found in the literature [42] , [43] , [44] , the corresponding column density is N H =2.3–3.3 × 10 20 cm −2 . This is comparable with the N H from X-ray spectral fitting. Next, we modelled the X-ray spectra in different pulsational phases. For this purpose, we sampled the observations for phases around the maximum ( φ =−0.1 to 0.2) and the minimum ( φ =0.4 to 0.8) of the X-ray light curve, respectively. These data are analysed in the same way as described above for the total exposure. The obtained results of the three temperature fits are compiled in Table 2 . Table 2 X-ray spectral properties of ξ 1 CMa. Full size table The table also gives the average plasma temperatures, ‹ kT ›, for the respective phases as mean values weighted with the emission measure. To estimate these mean values and their uncertainties, we perform a Monte Carlo evaluation for 10 5 values of the temperatures and the emission measures, randomized by their uncertainties and assuming normal and uncorrelated distributions. Then we take the mean and s.d. of the resulting values. These results are given in Table 2 . The spectral fits thus indicate that at the maximum of the pulsation cycle the average temperature is marginally higher (by about 40 eV or 500,000 K) than at minimum. The fluxes F X given in Table 2 are not corrected for the interstellar absorption and refer to the 0.2–10.0 keV energy range. During the pulsation cycle, the X-ray count rate changes by ≈10%. From the time between maximum and minimum of the light curve (2.5 h) one can estimate the cooling rate and use it to constrain the density of X-ray-emitting plasma. We computed cooling functions with the APEC code, and found that the observed cooling rate can only be achieved if the electron density is >≈3 × 10 8 cm −3 . According to our PoWR models for the cool wind of ξ 1 CMa, such high electron densities are encountered only close to the photospheric radius R * , and not farther than 1.05 R * . Assuming that the electron densities of the hot X-ray-emitting plasma are not higher than the densities of the ambient cool wind, the pulsed X-ray emission should originate from regions very close to the stellar photosphere. Otherwise, the timescale of X-ray variability would not be compatible with the cooling time. This estimate is based on the assumption of a smooth wind. In principle, one can envisage that the hot plasma density has strong local fluctuations, for example, it is enhanced at the magnetic equator [45] , [46] . In this case, sufficiently high density to allow for efficient cooling may be present farther out in the wind. Analysis of the high-resolution X-ray spectrum The high-resolution X-ray spectra of ξ 1 CMa obtained with the RGS1 and RGS2 spectrographs [29] are dominated by strong emission lines of metals. The spectrum obtained over the total exposure time and thus covering different pulsation phases can be well modelled by a thermal, optically thin plasma with temperatures that are consistent with those found from fitting the low-resolution spectra as described above (see Fig. 5 ). 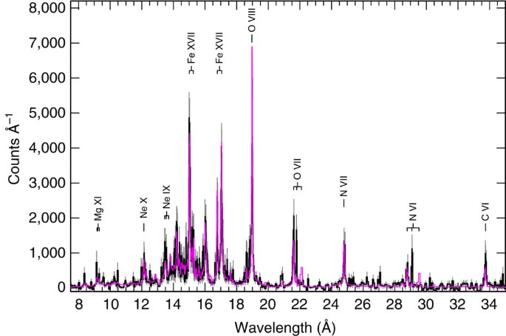Figure 5:High-resolution X-ray spectrum of ξ1CMa. Combined RGS spectrum of ξ1CMa integrated over the full exposure time is shown. Strong emission lines are identified. The best fit model is also shown (magenta line). Figure 5: High-resolution X-ray spectrum of ξ 1 CMa. Combined RGS spectrum of ξ 1 CMa integrated over the full exposure time is shown. Strong emission lines are identified. The best fit model is also shown (magenta line). Full size image The location of X-ray-emitting plasma can be constrained with the help of the lines from helium-like ions. These ions emit a group of three X-ray lines, consisting of a forbidden ( f ), an intercombination ( i ) and a resonance ( r ) transition—the so-called fir triplet. The ratio of fluxes G =( f + i )/ r is sensitive to the temperature, while the ratio of fluxes between the forbidden and the intercombination component, R = f / i , is sensitive to the electron density and the ultraviolet radiation field [47] : Here, φ denotes the photo-excitation rate from the term 2s 3 S to 2p 3 P, and N e is the electron density. The constants 0 , φ c and N c depend on atomic parameters and slightly on the electron temperature [48] . Most importantly, the photo-excitation rate φ ( r ) scales with the mean intensity of the radiation field at the wavelength of the f → r transition, which is typically in the ultraviolet. The fir triplets of Ne IX, O VII and N VI are present in the RGS spectrum of ξ 1 CMa, with the O VII triplet being the strongest one. Only in the O VII triplet, the forbidden line is marginally detected, while forbidden lines in Ne IX and N VI were not detected. We use the PoWR stellar atmosphere model to calculate the values of R ( r ) for Ne IX, O VII and N VI as a function of the radial location in the wind of ξ 1 CMa. The photo-excitation rates φ ( r ) are computed at each radius from the radiation intensity as provided by the PoWR model, which accounts not only for geometric dilution, but also for the diffuse radiation field. 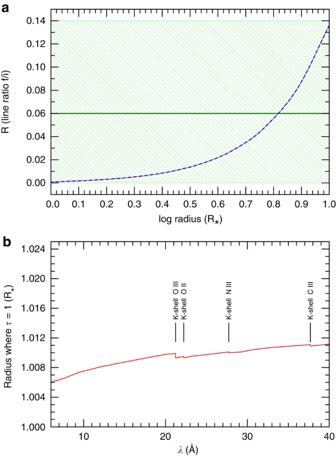Figure 6:Stellar wind model predictions for ξ1CMa. (a) Dependence of the line ratioR=f/ifor the O VIII lines as function of the radial location of the emitting plasma. On the basis of the PoWR model, the red curve accounts only for radiative de-population, while the almost identical blue curve also includes collisional processes under the assumption that the shocked plasma has the same density as the cool wind. The measured value is shown as a horizontal green line, with the green hatched area representing the 1σconfidence band of the measurement. (b) Radius (in units of the stellar radiusR*) where the cool wind from ξ1CMa becomes optically thin in dependence on the wavelength. The calculations were performed with the PoWR stellar atmosphere code (see text) with stellar parameters fromTable 1. Photoionization edges are identified. Figure 6a shows for the O VII triplet the predicted R ratio as a function of the radial location of the emitting plasma. From the spectrum integrated over the full exposure time, the best-fit value of the R ratio indicates a plasma location at ≈6 R * , while the 1 σ margins are consistent with any location between 1 R * and 10 R * . Figure 6: Stellar wind model predictions for ξ 1 CMa. ( a ) Dependence of the line ratio R = f / i for the O VIII lines as function of the radial location of the emitting plasma. On the basis of the PoWR model, the red curve accounts only for radiative de-population, while the almost identical blue curve also includes collisional processes under the assumption that the shocked plasma has the same density as the cool wind. The measured value is shown as a horizontal green line, with the green hatched area representing the 1 σ confidence band of the measurement. ( b ) Radius (in units of the stellar radius R * ) where the cool wind from ξ 1 CMa becomes optically thin in dependence on the wavelength. The calculations were performed with the PoWR stellar atmosphere code (see text) with stellar parameters from Table 1 . Photoionization edges are identified. Full size image X-ray line profiles formed in a rapidly expanding stellar wind would be Doppler broadened. These lines can appear characteristically blue-shifted and asymmetric, especially when there is significant absorption of the X-rays in the cool stellar wind [49] , [50] . To estimate the effects of wind absorption, we computed the radii at which the wind becomes optically thin for X-rays. The hot plasma is optically thin, and the X-rays are absorbed only in the cool wind via K-shell ionization of metals. As can be seen from Fig. 6b , the wind of ξ 1 CMa is optically thin for X-rays above ≈1.01 R * . To analyse the line shape, both RGS spectra were combined and line moments were calculated. Because of higher signal-to-noise ratio, the best-suited line for a detailed analysis is O VIII Lyα. This line is marginally broader than the instrumental response. The maximum wind velocity in ξ 1 CMa is ≈700 km s −1 . If X-ray lines were formed in a plasma moving with such velocity, the corresponding Doppler line broadening would be detectable in the high-resolution spectrum. Only for the O VIII Lyα line is a marginal blue-shift detected. Hence, the emitting plasma is not moving rapidly, and the attenuation of the X-rays by the cool wind is low. As a next step, we considered how the high-resolution spectrum varies between different pulsation phases (see Fig. 7 ). Surprisingly, the line ratios between the CNO elements change in different pulsation phases. Especially significant is the variability of the N VII Lyα resonance line (see Table 3 ). 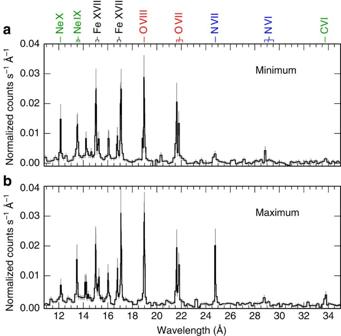Figure 7:Phase-dependent RGS spectra of ξ1CMa. (a) Combined high-resolution (RGS1+RGS2) spectrum in phase close to the pulsation minimumφ=0.6±0.2). (b) The same but in phase close to the pulsation maximum (φ=0.5±0.15). Strong emission lines are identified. The error bars correspond to 3σ. Figure 7: Phase-dependent RGS spectra of ξ 1 CMa. ( a ) Combined high-resolution (RGS1+RGS2) spectrum in phase close to the pulsation minimum φ =0.6±0.2). ( b ) The same but in phase close to the pulsation maximum ( φ =0.5±0.15). Strong emission lines are identified. The error bars correspond to 3 σ . Full size image Table 3 Photon flux in the N VII λ 24.78 Å line at different pulsation phases. Full size table It is unrealistic to assume that the observed changes of the N VII Lyα line strength with pulsational phase can be caused by a varying nitrogen abundance. It also seems unlikely that the N VII line variability is solely owing to changing densities and temperatures of the emitting plasma, since this would also affect other lines and line ratios. As an effect that selectively acts on the N VII Lyα line at λ =24.78 Å, we tentatively suggest varying absorption of the line emission by the cool wind component. According to our model (see Fig. 6b ), the cool wind becomes optically thick just close to the photosphere, the dominant opacity being due to K-shell ionization of N III ( ) [51] . However, at maximum an enhanced X-ray irradiation can shift the nitrogen ionization balance in the cool wind to higher stages. The K-shell edge of N V is already at a shorter wavelength ( ) than the N VII line. Thus, the attenuation of that line by the cool wind may be reduced at X-ray maximum, especially if the enhanced X-ray field is locally concentrated in the vicinity of confined X-ray production sites (such as shocks or hot spots on the stellar surface). It is generally assumed that X-ray emission from hot massive stars originates from plasma heated by hydrodynamic shocks in a radiatively driven stellar wind. The radiation-driven wind theory predicts that the mass-loss rate depends on the stellar parameters as where L bol is the stellar bolometric luminosity and α is a dimensionless number (which is about 2/3) representing the power-law exponent of the distribution function of line strength of the thousands of spectral lines driving the wind, and M eff ≈ M * for B-type stars [1] . During a pulsation cycle, the radius of ξ 1 CMa alters by 4% and its effective temperature by 3.6%. Recall that the luminosity is given by , where σ is Stefan–Boltzmann constant. With R * and T eff varying in anti-phase, the bolometric luminosity thus changes by ≈7% during a pulsation cycle. According to equation (2), the mass-loss rate may change by 10%, which is a similar amplitude as of the observed X-ray pulsations. According to the wind theory, the wind velocity scales with the escape velocity, that is, proportional to . Therefore it may also slightly change during the pulsation. The dynamical timescale for a stellar wind is the flow time . For ξ 1 CMa this time is about 2 h. Hence, the wind is, in principle, able to follow changes on the timescale of the pulsation period (5 h). From these considerations one might expect that the stellar pulsations lead to periodic variability of the wind parameters and, consequently, of the X-ray luminosity. However, while these scaling correlations are general, no X-ray pulsations from other massive stars have been detected so far. X-ray variability on the rotational timescale was observed in some stars, but its persistence and coherence is not established [36] , [52] , [53] , [54] . In X-ray pulsars associated with high-mass X-ray binaries, the pulsations are firmly attributed to the neutron stars. Previous to our detection, X-rays pulsations on the same timescale as stellar oscillations were not found in other β Cep-type variables [55] . Therefore, we believe that the general scaling correlations do not explain the observed X-ray properties of ξ 1 CMa. The analysis of the line ratio in the fir triplets, the estimates from cooling time and the tentative indications for the presence of the N IV K-shell absorption edge during the X-ray minimum consistently indicate that the X-ray-emitting plasma is located very close to the stellar photosphere. However, all models used in our analysis are spherically symmetric. Asymmetric wind structures may alter the interpretation. One may consider if the observed X-ray pulsations can be explained by geometrical occultation of the X-ray emission sites by an oscillating stellar disk. The stellar radius changes by 4% during oscillation. However, since the stellar disk can only block emission from the back hemisphere, occultation is not sufficient to explain the observed X-ray pulsations with 9% full amplitude. The new XMM-Newton observations of ξ 1 CMa may provide important insights into possible mechanisms of plasma heating. In β Cep-type variables the deposition of mechanical energy from the stellar pulsations can provide an additional heating [56] , [57] . However, in a study of a small sample of β Cep-type variables, no dependence of the X-ray luminosity on the pulsational period or amplitude was noticed [11] . In massive stars that possess large-scale magnetic fields, plasma heating is commonly explained by the magnetically confined wind shock mechanism [6] . This model predicts that the X-ray emission depends on mass-loss rate, wind velocity, stellar rotation and especially on the magnetic field strength [11] , [46] , [58] , [61] . To check this prediction, we compare our data with the XMM-Newton observations of similar quality that are available for two other magnetic β Cep-type stars, β Cen (B1III) and β Cep (B2V) [25] , [55] , [59] , [60] , [62] . These stars have roughly the same mass-loss rate and wind velocity, but ξ 1 CMa has a much stronger magnetic field. The observations now reveal that the X-ray spectra and forbidden-to-intercombination line ratios are similar in all these stars, the only significant difference being that the X-rays from ξ 1 CMa pulsate. It is illuminating to compare ξ 1 CMa with the degenerate X-ray pulsars, namely white dwarfs and neutron stars [63] , [64] , [65] . Some neutron star X-ray pulsars have a thermal component in their X-ray spectra, which is explained as originating from their atmosphere [66] . However, the effective temperatures of our B-type star is lower by an order of magnitude. Therefore, the mechanism of its thermal X-ray emission must be principally different. The first observations of stellar atmospheric pulsational phenomena in the X-ray band were reported from the hot, helium-rich, pulsating degenerate object PG 1159-035 (ref. 67 ). The X-ray pulsations arise from the photosphere of PG 1159-035, which has T eff >100,000 K and is thus significantly hotter than ξ 1 CMa. We rule out that the X-ray pulsations observed in ξ 1 CMa may be explained by an oscillating stellar photosphere—the stellar temperature is not hot enough to contribute even to the softest X-ray band. Rapid quasi-periodic oscillations in X-ray light were detected in some bursting magnetic neutron stars (for example, SGR 1806-20 and SGR 1900+14). Those oscillations may be interpreted in terms of the coupling of toroidal seismic modes with Alfvén waves propagating along magnetospheric field lines. They provide evidence that the vibration modes of the neutron star crust excited by strong flares are manifested in the X-ray light [68] , [69] , [70] . Albeit the energetics in non-degenerate B-type star are vastly different from those in the neutron star magnetars, it is important to use the analogies and investigate in future work the possible coupling of radial stellar oscillations with Alfvén waves in ξ 1 CMa. The properties that make ξ 1 CMa distinct from other β Cep-type variables are the supersonic speed of the pulsating photosphere, the high strength of the star’s magnetic field and the absence of non-radial modes in the stellar oscillations. We suggest that a successful explanatory model must take these ingredients into account in order to understand the X-ray emission and its periodic modulations observed in ξ 1 CMa. To summarize, we detect pulsations of the X-ray flux from ξ 1 CMa in phase with optical pulsations but with larger amplitude. The X-ray light curves are similar in different energy bands. There are tentative indications that changes of the X-ray emission are due to the plasma heating and cooling—from the spectral analysis, somewhat higher temperatures are deduced at X-ray maximum as compared with X-ray minimum. The X-ray-emitting plasma is located close to the photosphere, as follows from the cooling rate and from the analysis of line ratios in He-like ions. This discovery of X-ray pulsations from a non-degenerate, massive star will stimulate theoretical considerations for the physical processes operating in magnetized stellar winds. So far, the mechanism by which the X-rays are affected by the stellar pulsations remains enigmatic. How to cite this article: Oskinova, L. M. et al. Discovery of X-ray pulsations from a massive star. Nat. Commun. 5:4024 doi: 10.1038/ncomms5024 (2014).